Nrf2 reduces levels of phosphorylated tau protein by inducing autophagy adaptor protein NDP52 Nuclear factor erythroid 2-related factor 2 (Nrf2) is a pivotal transcription factor in the defence against oxidative stress. Here we provide evidence that activation of the Nrf2 pathway reduces the levels of phosphorylated tau by induction of an autophagy adaptor protein NDP52 (also known as CALCOCO2) in neurons. The expression of NDP52, which we show has three antioxidant response elements (AREs) in its promoter region, is strongly induced by Nrf2, and its overexpression facilitates clearance of phosphorylated tau in the presence of an autophagy stimulator. In Nrf2 -knockout mice, phosphorylated and sarkosyl-insoluble tau accumulates in the brains concurrent with decreased levels of NDP52. Moreover, NDP52 associates with phosphorylated tau from brain cortical samples of Alzheimer disease cases, and the amount of phosphorylated tau in sarkosyl-insoluble fractions is inversely proportional to that of NDP52. These results suggest that NDP52 plays a key role in autophagy-mediated degradation of phosphorylated tau in vivo . In Alzheimer disease (AD), tau becomes aberrantly phosphorylated and oligomerized which likely contributes to neuronal dysfunction and death [1] , [2] , [3] . The mechanism involved in clearing pathological, phosphorylated tau has not yet been fully defined. Given that tau plays a central role in the pathogenesis of AD [2] , [3] , there is a growing interest in understanding the processes by which pathological, phosphorylated tau is removed from neurons and subsequently developing interventions that result in the selective removal of the pathological tau as a therapeutic approach for the treatment of AD [2] , [4] . To date, several reports have suggested that misfolded or phosphorylated tau could be degraded through the proteasome [5] , [6] , [7] , [8] . On the other hand, some studies found that tau was not degraded by the proteasome, and unexpectedly observed decreases in the levels of tau in the presence of proteasome inhibitors [9] , [10] . In addition to degradation by the proteasome, several groups have presented data indicating that tau can be turned over by the autophagy–lysosome pathway [11] , [12] , [13] , [14] , [15] , [16] , [17] . The triage process directing specific forms of tau to a given degradation pathway is not completely understood and is an area of interest. A family of autophagy adaptor proteins that contain LC3-interacting regions (LIRs) has been identified and include p62/sequestosome 1 (SQSTM1), neighbour of BRCA1 gene 1 (NBR1) and nuclear dot protein 52 (NDP52) [18] , [19] . The most well-studied member of this group is p62/SQSTM1, a multifunctional protein that acts as a scaffold for signalling protein complexes as well as being an adaptor for protein trafficking, aggregation and degradation [20] . p62/SQSTM1 also plays an important role in regulating the nuclear factor erythroid 2-related factor 2 (Nrf2) pathway [21] , as well as being upregulated by Nrf2 (ref. 22 ). Genetic inactivation of p62/SQSTM1 in mice leads to an accumulation of hyperphosphorylated tau [23] . NBR1 was shown to be involved in the autophagy targeting of ubiquitylated substrates [24] and defective ribosomal products [25] , and co-localized with phosphorylated tau together with p62/SQSTM1 in the muscle fibre aggregates of sporadic inclusion-body myositis [26] . NDP52 has been identified primarily in peripheral tissues as an innate immune autophagy receptor for ubiquitylated bacteria, thus coordinating their destruction by the autophagy pathway [27] , [28] . NDP52 also functions as an autophagic adaptor for the selective degradation of TRIF (Toll/IL-1 receptor homology domain-containing adaptor inducing interferon-β) and TRAF6 (tumour necrosis-receptor-associated factor 6) in the periphery [29] . Recently, it was suggested that NDP52 participates in autophagosome maturation by docking with myosin VI together with TRAF 6 binding protein (T6BP) and optineurin [30] . However, a biological role for NDP52 in neurons or in mediating the degradation of tau has not been examined. Oxidative stress has been considered as one of the early pathogenic events during disease progression in the brains of AD patients [31] . One of the defence mechanisms against oxidative stress as well as other stressors is the activation of the Nrf2 pathway [32] . Nrf2 acts by binding to the consensus antioxidant response element (ARE) sequence following heterodimerization with Maf, leading to the expression of genes involved in protein degradation like p62/STSQM1 (ref. 22 ), as well as cytoprotective genes including haeme oxygenase 1, NAD(P)H:quinine oxidoreductase 1 and glutathione peroxidase [32] . Although activation of Nrf2 improved learning and memory retention in a mouse model of AD [33] , [34] , there is no study on its role in the clearance of pathological, phosphorylated tau. Here we show that in Nrf2 -knockout mice the levels of phosphorylated tau and the levels of sarkosyl-insoluble tau are increased. We also demonstrate that NDP52 is a Nrf2 responsive gene and a major, downstream facilitator of Nrf2-mediated phosphorylated tau degradation by autophagy. Nrf2 activation promotes degradation of phosphorylated tau To examine whether Nrf2 is involved in the degradation of phosphorylated tau, we examined the levels of phosphorylated tau in the hippocampal tissues of Nrf2 -knockout (−/−) mice. As shown in Fig. 1a,b and Supplementary Fig. 1 , 2.9- and 2.7-fold increases of tau phosphorylated at Ser262/Ser356 [12E8] and at Ser396/Ser404 [PHF1], respectively, were observed in Nrf2 (−/−) mice in comparison with wild-type mice. In addition, the level of total tau also showed a 1.8- or 2.1-fold increase by the use of a polyclonal tau or the Tau5 antibody, respectively. When the presence of phosphorylated tau in the hippocampal region was immunohistochemically evaluated, phosphorylated tau staining with the 12E8 or PHF1 antibodies was readily detected in the hippocampal region of Nrf2 (−/−) mice, whereas almost none was apparent in wild-type mice ( Fig. 1c,d ). Further, the amount of sarkosyl-insoluble tau was 5.3-fold increased in Nrf2 (−/−) mice compared with wild-type mice ( Fig. 2 ). These results suggest that Nrf2 is involved in the degradation of pathologic, phosphorylated tau. 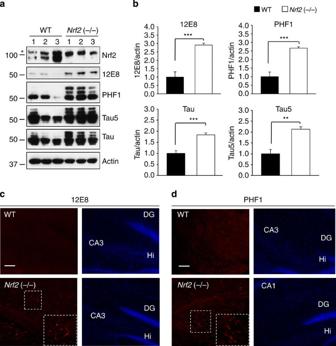Figure 1:Phosphorylated tau accumulates in the hippocampus ofNrf2(−/−) mice. (a) Hippocampal tissues obtained fromNrf2(−/−) (6 months old, one male and two female) or wild-type (WT) (11 months old, two male and one female) mice were immunoblotted with a Nrf2 antibody, 12E8, PHF1, a monoclonal to total tau (Tau5) or a polyclonal to total tau (Tau) antibody. The asterisk to the left of the Nrf2 blot designates the position at which a nonspecific band migrated. The relative molecular masses (kDa) are indicated to the left of each blot. (b) Bar graphs represent the relative optical density of phosphorylated or total tau in the hippocampal tissues.n=6 (These data are based on the mouse hippocampi immunoblotted inSupplementary Fig. 1). Data shown are mean±s.e. and were analysed using Student’st-test. (**P<0.01; ***P<0.001) (c,d) Left panels show brain sections stained for tau phosphorylated at Ser262/Ser356 (12E8) (c) and Ser396/Ser404 (PHF1) (d). The area of delineated by dotted lines is enlarged and shown in the right corner of the image. Right panels shows the same slice stained with 4',6-diamidino-2-phenylindole. Scale bar, 50 μm. DG, dentate gyrus; Hi, dentate hilar area. Figure 1: Phosphorylated tau accumulates in the hippocampus of Nrf2 (−/− ) mice. ( a ) Hippocampal tissues obtained from Nrf2 (−/−) (6 months old, one male and two female) or wild-type (WT) (11 months old, two male and one female) mice were immunoblotted with a Nrf2 antibody, 12E8, PHF1, a monoclonal to total tau (Tau5) or a polyclonal to total tau (Tau) antibody. The asterisk to the left of the Nrf2 blot designates the position at which a nonspecific band migrated. The relative molecular masses (kDa) are indicated to the left of each blot. ( b ) Bar graphs represent the relative optical density of phosphorylated or total tau in the hippocampal tissues. n =6 (These data are based on the mouse hippocampi immunoblotted in Supplementary Fig. 1 ). Data shown are mean±s.e. and were analysed using Student’s t -test. (** P <0.01; *** P <0.001) ( c , d ) Left panels show brain sections stained for tau phosphorylated at Ser262/Ser356 (12E8) ( c ) and Ser396/Ser404 (PHF1) ( d ). The area of delineated by dotted lines is enlarged and shown in the right corner of the image. Right panels shows the same slice stained with 4',6-diamidino-2-phenylindole. Scale bar, 50 μm. DG, dentate gyrus; Hi, dentate hilar area. 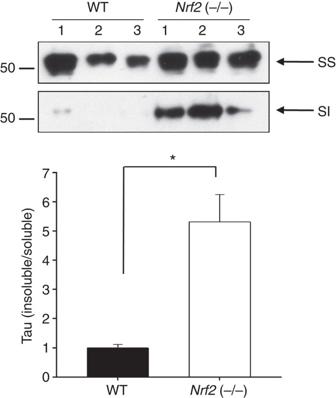Figure 2:Sarkosyl-insoluble tau accumulates in the hippocampus ofNrf2(−/−) mice. Brain cortical tissue obtained fromNrf2(−/−) (6 months old, one male and two female) or wild-type (11 months old, two male and one female) mice were separated into sarkosyl-soluble (SS) and insoluble (SI) fractions as described in the Methods. The level of total tau was analysed by immunoblotting using a monoclonal antibody to total tau (Tau5). The relative molecular masses (kDa) are indicated to the left of each blot. Bar graph represents the relative optical density of sarkosyl-insoluble tau normalized with that of sarkosyl-soluble tau.n=3. Data shown are mean±s.e. and were analysed using Student’st-test. (*P<0.05). Full size image Figure 2: Sarkosyl-insoluble tau accumulates in the hippocampus of Nrf2 (−/− ) mice. Brain cortical tissue obtained from Nrf2 (−/−) (6 months old, one male and two female) or wild-type (11 months old, two male and one female) mice were separated into sarkosyl-soluble (SS) and insoluble (SI) fractions as described in the Methods. The level of total tau was analysed by immunoblotting using a monoclonal antibody to total tau (Tau5). The relative molecular masses (kDa) are indicated to the left of each blot. Bar graph represents the relative optical density of sarkosyl-insoluble tau normalized with that of sarkosyl-soluble tau. n =3. Data shown are mean±s.e. and were analysed using Student’s t -test. (* P <0.05). Full size image To further investigate whether Nrf2 activity is involved in the degradation of phosphorylated tau, primary rat cortical neurons and immortalized CN1.4 mouse cortical cells that inducibly express wild-type tau [14] were treated with sulforaphane (10 μM, SFN), an Nrf2 activator ( Supplementary Fig. 2a,b ). Twenty-four hours after treatment with SFN the levels of tau phosphorylated at Ser262/Ser356 [12E8] were reduced 30 and 70% in primary cortical neurons and CN1.4 mouse cortical cells, respectively. In the case of tau phosphorylated at Ser396/Ser404 [PHF1], 50 and 43% reductions were observed, respectively ( Fig. 3 ). Treatment with 10 μM of SFN did not affect the viability of neurons ( Supplementary Fig. 2d,e ), indicating that the reduction of phosphorylated tau was not due to increased cell death in the presence of SFN. In addition, when primary rat cortical neurons were treated with 50 μM tert -butylhydroquinone (tBHQ), another Nrf2 activator ( Supplementary Fig. 2c ), a significant reduction of tau phosphorylated at Ser262/Ser356 [12E8] and Ser396/Ser404 [PHF1] was also observed as shown in Supplementary Fig. 3a–c . Thus, these results suggest that Nrf2 activation facilitates the degradation of phosphorylated tau. 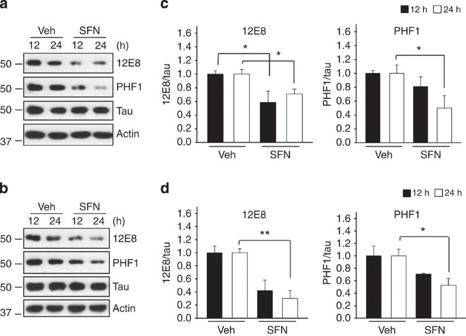Figure 3: Nrf2 activation enhances the degradation of phosphorylated tau in neurons. (a) Primary cortical neurons (DIV 5) were treated with SFN (10 μM, SFN) for 12 or 24 h. (b) Stably transfected CN1.4 cortical neurons were maintained in the presence of doxycycline (1 μg ml−1) to induce the expression of tau for 24 h, and subsequently treated with SFN for 12 or 24 h. The levels of tau phosphorylated at Ser262/Ser356 and Ser396/Ser404 were analysed by immunoblotting using the 12E8 and PHF1 antibodies, respectively. Tau was detected with a polyclonal phospho-independent tau antibody (Tau). The relative molecular masses (kDa) are indicated to the left of each blot. (c,d) Bar graphs represent the relative optical density of phosphorylated tau normalized with that of total tau. Data shown are mean±s.e. of three independent experiments and were analysed using Student’st-test. (*P<0.05; **P<0.01). Figure 3: Nrf2 activation enhances the degradation of phosphorylated tau in neurons. ( a ) Primary cortical neurons (DIV 5) were treated with SFN (10 μM, SFN) for 12 or 24 h. ( b ) Stably transfected CN1.4 cortical neurons were maintained in the presence of doxycycline (1 μg ml −1 ) to induce the expression of tau for 24 h, and subsequently treated with SFN for 12 or 24 h. The levels of tau phosphorylated at Ser262/Ser356 and Ser396/Ser404 were analysed by immunoblotting using the 12E8 and PHF1 antibodies, respectively. Tau was detected with a polyclonal phospho-independent tau antibody (Tau). The relative molecular masses (kDa) are indicated to the left of each blot. ( c , d ) Bar graphs represent the relative optical density of phosphorylated tau normalized with that of total tau. Data shown are mean±s.e. of three independent experiments and were analysed using Student’s t -test. (* P <0.05; ** P <0.01). Full size image Tau phosphotransferases are not different in Nrf2 (−/−) mice The Ser/Thr-Pro sites of tau have been proposed to be phosphorylated by such kinases as cyclin-dependent kinase 5, glycogen synthase kinase 3β and extracellular signal-regulated kinase 2, while the KXGS motif (the 12E8 epitope) in the microtubule-binding domains is probably phosphorylated by microtubule affinity regulating kinases [1] . Given the results, it is possible that the increased levels of phosphorylated tau could result from increased kinase activity in Nrf2 (−/−) mice. Thus, we performed in vitro kinase assays using mouse brain lysates and found there was no significant difference in kinase activity between Nrf2 (−/−) and wild-type mice ( Fig. 4a and Supplementary Fig. 4 ). It can also be speculated that in Nrf2 (−/−) mice there may be decreased activity of protein phosphatase 2A (PP2A), since PP2A is known to be the primary phosphatase involved in the dephosphorylation of tau [35] , [36] . When the activity of protein phosphatases was assayed using mouse brain lysates, there was no difference in the activity of PP2A, between Nrf2 (−/−) and wild-type mice ( Fig. 4b ). These results strongly support the conclusion that the increased levels of phosphorylated tau in Nrf2 (−/−) mouse brain does not result from alterations in the activities of kinases or phosphatases. 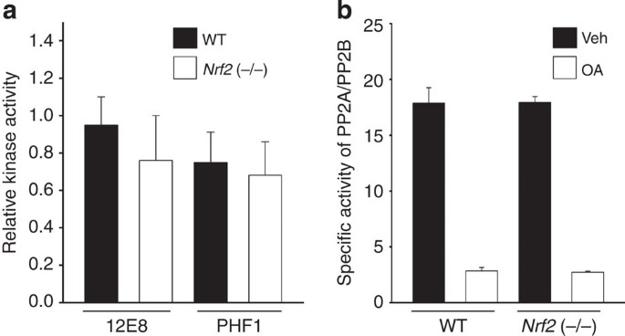Figure 4:There is no significant difference in tau kinase and phosphatase activities between wild-type andNrf2(−/−) mice. Mouse brains were obtained from wild-type (11 months old, one male; 5 months old, one female; 12 months old, two female) andNrf2(−/−) (10 months old, two male and two female) mice. (a)Mouse brain tissues were homogenized in the lysis buffer, and 10 μg of lysates was incubated with 2 μg of GST-tau protein at 37 °C for 30 min in the presence or absence of 1 mM ATP. The levels of tau phosphorylated at Ser262/Ser356 and Ser396/Ser404 were analysed by immunoblotting using a 12E8 and PHF1 antibodies, respectively. GST-tau was detected with a monoclonal GST antibody (GST-tau;Supplementary Fig. 4). Bar graph of the relative optical density of phosphorylated tau normalized to actin. Data shown are mean±s.e. of duplicated independent experiments and were analysed using Student’st-test. (b) Mouse brain tissues were homogenized in the phosphatase storage buffer, and phosphatase activity in the lysates was quantified using the serine/threonine phosphatase assay system (Promega) by measuring the dephosphorylation of a phosphopeptide, RRA(pT)VA in the presence or absence of okadaic acid (OA, 20 nM). PP2A activity was defined as the activity inhibited by the addition of OA to the phosphatase reaction mixture.n=4. Data shown are mean±s.e. of three independent experiments and were analysed using Student’st-test. Figure 4: There is no significant difference in tau kinase and phosphatase activities between wild-type and Nrf2 (−/− ) mice. Mouse brains were obtained from wild-type (11 months old, one male; 5 months old, one female; 12 months old, two female) and Nrf2 (−/−) (10 months old, two male and two female) mice. ( a )Mouse brain tissues were homogenized in the lysis buffer, and 10 μg of lysates was incubated with 2 μg of GST-tau protein at 37 °C for 30 min in the presence or absence of 1 mM ATP. The levels of tau phosphorylated at Ser262/Ser356 and Ser396/Ser404 were analysed by immunoblotting using a 12E8 and PHF1 antibodies, respectively. GST-tau was detected with a monoclonal GST antibody (GST-tau; Supplementary Fig. 4 ). Bar graph of the relative optical density of phosphorylated tau normalized to actin. Data shown are mean±s.e. of duplicated independent experiments and were analysed using Student’s t -test. ( b ) Mouse brain tissues were homogenized in the phosphatase storage buffer, and phosphatase activity in the lysates was quantified using the serine/threonine phosphatase assay system (Promega) by measuring the dephosphorylation of a phosphopeptide, RRA(pT)VA in the presence or absence of okadaic acid (OA, 20 nM). PP2A activity was defined as the activity inhibited by the addition of OA to the phosphatase reaction mixture. n =4. Data shown are mean±s.e. of three independent experiments and were analysed using Student’s t -test. Full size image Autophagy mediates the degradation of phosphorylated tau To investigate the contribution of the proteasome and autophagy pathways to the degradation of phosphorylated tau, we examined the levels of phosphorylated tau in CN1.4 cortical cells [14] using inhibitors. Following withdrawal of doxycycline, tau (and phospho-tau) levels decreased as expected. Treatment with the autophagy inhibitor, 3-methyladenine (3-MA, 10 mM) for 24 h following the withdrawal of doxycycline inhibited the degradation of phosphorylated tau and total tau ( Fig. 5a ). In contrast, treatment with the proteasome inhibitors epoxomicin (12.5 nM) or MG132 (7 μM) increased phosphorylated tau degradation ( Fig. 5a ). These data are in agreement with a recent study that showed proteasome inhibition in primary cortical neurons increased autophagy and tau clearance, and that 3-MA reduces tau clearance [15] . Further, addition of chloroquine (CQ, 50 μM) or bafilomycin A1 (10 nM) [37] to media devoid of doxycycline attenuated the degradation of phosphorylated tau and total tau ( Fig. 5b ). Also, the knockdown of beclin-1, a key molecule of the autophagy pathway, using short interfering RNA (siRNA) resulted in an accumulation of tau ( Fig. 5c ). Interestingly, SFN causes an increase in autophagy in neurons ( Supplementary Figs 5 and 6 ); thus, the SFN (10 μM) -induced reduction in phosphorylated tau levels ( Fig. 3 ) is likely due to increased autophagic clearance. Indeed, the SFN-induced degradation of tau was significantly attenuated by CQ ( Fig. 5d,e ). These data strongly indicate that the autophagy pathway plays a major role in the degradation of phosphorylated tau. 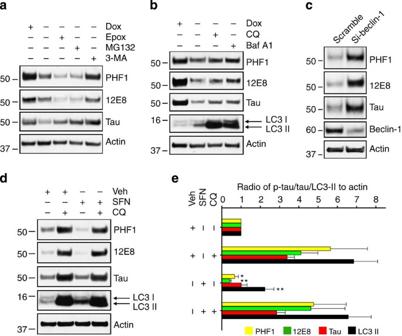Figure 5: Autophagy contributes to tau clearance in neuronal cells. CN1.4 mouse cortical cells stably expressing inducible tau were treated with doxycycline (Dox, 1 μg ml−1) for 24 h. On the next day (a), the cells were washed twice with PBS and the media were replaced with Dox-deficient media with either vehicle, epoxomicin (12.5 nM, Epox), MG132 (7 μM) or 3-methyladenine (10 mM, 3-MA) for 24 h. (b) Cells were treated with either chloroquine (50 μM, CQ) or bafilomycin A1 (10 nM, Baf A1) for 24 h. Samples in first lane were from cells maintained in the presence of Dox without medium exchange. (c) HEK293-TN cells were co-transfected with the plasmid expressing tau together either with siRNA of beclin-1 or scramble RNA as a control, which was kept for 48 h. (d) Stably transfected CN1.4 cortical cells were maintained in the presence of Dox (1 μg ml−1) to induce the expression of tau for 24 h, and subsequently treated with SFN (10 μM) for 12 h. The culture medium was exchanged for fresh media containing Dox (1 μg ml−1) but no SFN after washing with PBS. The cells were then incubated for an additional 18 h in the absence or presence of CQ (50 μM). The levels of tau phosphorylated at Ser262/Ser356 and Ser396/Ser404 were analysed by immunoblotting using the 12E8 and PHF1 antibodies, respectively. Tau, beclin-1 and LC3 were detected with the appropriate polyclonal antibodies. The relative molecular masses (kDa) are indicated to the left of each blot. (e) Bar graphs represent the relative optical density of phosphorylated tau, tau or LC3-II normalized with that of actin.n=4. Data shown are mean±s.e. and were analysed using Student’st-test. (*P<0.05; **P<0.01). Figure 5: Autophagy contributes to tau clearance in neuronal cells. CN1.4 mouse cortical cells stably expressing inducible tau were treated with doxycycline (Dox, 1 μg ml −1 ) for 24 h. On the next day ( a ), the cells were washed twice with PBS and the media were replaced with Dox-deficient media with either vehicle, epoxomicin (12.5 nM, Epox), MG132 (7 μM) or 3-methyladenine (10 mM, 3-MA) for 24 h. ( b ) Cells were treated with either chloroquine (50 μM, CQ) or bafilomycin A1 (10 nM, Baf A1) for 24 h. Samples in first lane were from cells maintained in the presence of Dox without medium exchange. ( c ) HEK293-TN cells were co-transfected with the plasmid expressing tau together either with siRNA of beclin-1 or scramble RNA as a control, which was kept for 48 h. ( d ) Stably transfected CN1.4 cortical cells were maintained in the presence of Dox (1 μg ml −1 ) to induce the expression of tau for 24 h, and subsequently treated with SFN (10 μM) for 12 h. The culture medium was exchanged for fresh media containing Dox (1 μg ml −1 ) but no SFN after washing with PBS. The cells were then incubated for an additional 18 h in the absence or presence of CQ (50 μM). The levels of tau phosphorylated at Ser262/Ser356 and Ser396/Ser404 were analysed by immunoblotting using the 12E8 and PHF1 antibodies, respectively. Tau, beclin-1 and LC3 were detected with the appropriate polyclonal antibodies. The relative molecular masses (kDa) are indicated to the left of each blot. ( e ) Bar graphs represent the relative optical density of phosphorylated tau, tau or LC3-II normalized with that of actin. n =4. Data shown are mean±s.e. and were analysed using Student’s t -test. (* P <0.05; ** P <0.01). Full size image NDP52 expression is dependent on Nrf2 To elucidate the downstream molecules involved in the Nrf2-mediated turnover of phosphorylated tau, we determined the transcript levels of the autophagy adaptor proteins p62/SQSTM1, NBR1 and NDP52 (refs 18 , 19 ) using quantitative real-time PCR (qRT–PCR) in the primary cortical neurons and CN1.4 cortical cells [14] following treatment with SFN (10 μM) for 12 h. As shown in Fig. 6a and Supplementary Fig. 7 , a 1.7-fold increase of p62/SQSTM1 messenger RNA was observed in the CN1.4 cortical cells, but not in the primary cultured neurons. NBR1 mRNA was not affected by SFN treatment in both cell types. However, in the case of NDP52 mRNA, expression was induced 2.4- and 2.6-fold in the primary cultured neurons and the CN1.4 mouse cortical cells, respectively, following SFN treatment. Analysis of the transcript levels of these genes in the hippocampal tissues of Nrf2 (−/−) mice revealed that p62/SQSTM1 mRNA was significantly decreased 1.9-fold, compared with wild-type mice. By contrast, the decrease of NDP52 mRNA in the Nrf2 (−/−) mice was much more dramatic, as the level was 7.8-fold lower than in wild-type mice. This decrease was even greater than the decrease in the mRNA for haeme oxygenase 1 (approximately threefold), a well-known Nrf2 downstream gene ( Fig. 6b ). Protein levels of p62/SQSTM1 and NDP52, which showed a significant difference in the mRNA levels between Nrf2 (−/−) and wild-type mice, were also determined. In line with the results of the qRT–PCR, NDP52 protein was scarcely detected in the hippocampal tissues of Nrf2 (−/−) mice compared with those of wild-type mice ( Fig. 6c and Supplementary Fig. 8c,d ); however, no differences were observed in the protein levels of p62/SQSTM1 despite its decrease at the mRNA level ( Fig. 6c ). 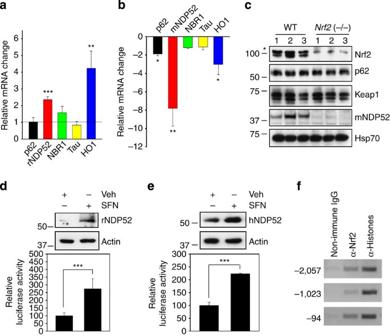Figure 6:NDP52 is induced by Nrf2 activation and its expression is significantly reduced inNrf2(−/−) mice. (a) Primary cortical neurons (DIV 5) were treated with SFN (10 μM) for 12 h, and the relative mRNA level of each gene was compared with that of cells not treated with SFN using qRT–PCR. (b) In hippocampal tissues fromNrf2(−/−) (5 months old, one male; 11 months old, one female; 5 months old, one female; 12 months old, three female) or wild-type (10 months old, four male and two female) mice, the relative mRNA level of each gene compared with that of wild-type mice.n=6. (c) The levels of p62/SQSTM1, Keap1, mouse NDP52 (mNDP52) and Hsp70 inNrf2(−/−) or wild-type mice were examined by immunoblotting. The asterisk on the Nrf2 panel indicates a nonspecific band. (d,e: upper panel) Primary cortical neurons (DIV 5) (d) and SH-SY5Y cells (e) were treated with SFN for 24 h, and the expression levels of rat and human NDP52 (rNDP52 and hNDP52) examined by immunoblotting using anti-NDP52 antibody. The relative molecular masses (kDa) are indicated to the left of each blot. (d,e: low panel) Primary cortical neurons (DIV 5) (d) and SH-SY5Y cells (e) transiently transfected with the pGL4.14/human NDP52 promoter (2,173 bp) luciferase reporter plasmid were treated with SFN for 24 h, and assayed for the luciferase activity. (f) SH-SY5Y cells were treated with SFN for 12 h, and cell lysates were used for the ChIP assay using anti-Nrf2 antibody as described in the Methods. Data shown are mean±s.e. and were analysed using Student’st-test. (*P<0.05; **P<0.01; ***P<0.001). Figure 6: NDP52 is induced by Nrf2 activation and its expression is significantly reduced in Nrf2 (−/− ) mice. ( a ) Primary cortical neurons (DIV 5) were treated with SFN (10 μM) for 12 h, and the relative mRNA level of each gene was compared with that of cells not treated with SFN using qRT–PCR. ( b ) In hippocampal tissues from Nrf2 (−/−) (5 months old, one male; 11 months old, one female; 5 months old, one female; 12 months old, three female) or wild-type (10 months old, four male and two female) mice, the relative mRNA level of each gene compared with that of wild-type mice. n =6. ( c ) The levels of p62/SQSTM1, Keap1, mouse NDP52 (mNDP52) and Hsp70 in Nrf2 (−/−) or wild-type mice were examined by immunoblotting. The asterisk on the Nrf2 panel indicates a nonspecific band. ( d , e : upper panel) Primary cortical neurons (DIV 5) ( d ) and SH-SY5Y cells ( e ) were treated with SFN for 24 h, and the expression levels of rat and human NDP52 (rNDP52 and hNDP52) examined by immunoblotting using anti-NDP52 antibody. The relative molecular masses (kDa) are indicated to the left of each blot. ( d , e : low panel) Primary cortical neurons (DIV 5) ( d ) and SH-SY5Y cells ( e ) transiently transfected with the pGL4.14/human NDP52 promoter (2,173 bp) luciferase reporter plasmid were treated with SFN for 24 h, and assayed for the luciferase activity. ( f ) SH-SY5Y cells were treated with SFN for 12 h, and cell lysates were used for the ChIP assay using anti-Nrf2 antibody as described in the Methods. Data shown are mean±s.e. and were analysed using Student’s t -test. (* P <0.05; ** P <0.01; *** P <0.001). Full size image If the transcription of NDP52 is dependent on Nrf2 activation, there should be conserved AREs for Nrf2 in the promoter region of human NDP52. Interestingly, five putative, consensus cis -acting ARE elements were identified in the promoter DNA sequence ( Fig. 7a ). Therefore, we cloned the promoter region (2,137 bps) of human NDP52 gene from human genomic DNA. The protein levels of NDP52, as well as the luciferase activities of human NDP52 promoter, were significantly induced in both primary cultured neurons and SH-SY5Y cells in response to SFN (10 μM) treatment ( Fig. 6d,e ). In addition, the protein level of NDP52 increased in SH-SY5Y cells in response to tBHQ (50 μM) treatment ( Supplementary Fig. 3d ). To identify which of the consensus ARE sites in the NDP52 promoter are functional, we made several site-directed or deleted mutants of the putative ARE sites such that the Nrf2/Maf complex would be unable to bind. The luciferase activity of NDP52 promoter was abolished with the deletion of between −450 and +1 (HindIII), indicating this region is very important in the basal transcription of NDP52 gene ( Fig. 7b ). Nrf2-induced luciferase activity was completely abolished only when the three functional ARE sites (−2,057, −1,023 and −94) in the NDP52 promoter were mutated ( Fig. 7c,d ). The direct binding of Nrf2 to these ARE sites in vivo was confirmed with a chromatin immunoprecipitation (ChIP) assay ( Fig. 6f ). Together, the results suggest that the expression of NDP52 is strongly dependent on the activity of Nrf2 and mediated by the direct binding of Nrf2 to its promoter. 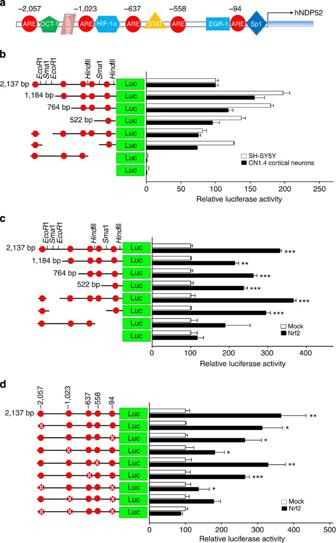Figure 7:There are three functional AREcis-elements in the human NDP52 promoter. (a) Diagram shows five putative AREcis-acting elements in human NDP52 promoter region (2,137 bp). Red ellipsoids indicate the putative AREcis-acting elements. (b–d) The mutant forms of pGL4.14-Luc reporter plasmid with the human NDP52 promoter gene were prepared by digestion with specific restriction enzymes (for example, HindIII, SmaI or EcoRI) by cloning of specific regions following PCR amplification or with the QuikChange site-directed mutagenesis kit (Agilent Technologies). (b) CN1.4 cortical cells and SH-SY5Y cells were transiently transfected with the reporter plasmids with the human NDP52 promoter (2,317 bp or deleted mutants), and luciferase activity was assayed 24 h after transfection. (c) SH-SY5Y cells were co-transfected with the reporter plasmids with human NDP52 promoter (wild or deleted mutants) along with either the mock plasmid (pcDNA3.1) or the plasmid expressing Nrf2, and the luciferase activity was assayed 24 h after transfection. (d) SH-SY5Y cells were transiently co-transfected with the reporter plasmids with human NDP52 promoter or its mutant plasmid in which the putative ARE sequence was site-directly mutated (X), together with the mock plasmid (pcDNA3.1) or the plasmid expressing human Nrf2. The luciferase activity was assayed after 24 h. The induced luciferase activity with co-expression with Nrf2 was not observed in a mutant NDP52 promoter in which all three ARE sites (−2,057, −1,023 and −94) were site-directly mutated, indicating these three sites of five AREcis-acting elements are functional. Data shown are mean±s.d. of three independent experiments and were analysed using Student’st-test. (*P<0.05; **P<0.01; ***P<0.001). Figure 7: There are three functional ARE cis -elements in the human NDP52 promoter. ( a ) Diagram shows five putative ARE cis -acting elements in human NDP52 promoter region (2,137 bp). Red ellipsoids indicate the putative ARE cis -acting elements. ( b – d ) The mutant forms of pGL4.14-Luc reporter plasmid with the human NDP52 promoter gene were prepared by digestion with specific restriction enzymes (for example, HindIII, SmaI or EcoRI) by cloning of specific regions following PCR amplification or with the QuikChange site-directed mutagenesis kit (Agilent Technologies). ( b ) CN1.4 cortical cells and SH-SY5Y cells were transiently transfected with the reporter plasmids with the human NDP52 promoter (2,317 bp or deleted mutants), and luciferase activity was assayed 24 h after transfection. ( c ) SH-SY5Y cells were co-transfected with the reporter plasmids with human NDP52 promoter (wild or deleted mutants) along with either the mock plasmid (pcDNA3.1) or the plasmid expressing Nrf2, and the luciferase activity was assayed 24 h after transfection. ( d ) SH-SY5Y cells were transiently co-transfected with the reporter plasmids with human NDP52 promoter or its mutant plasmid in which the putative ARE sequence was site-directly mutated (X), together with the mock plasmid (pcDNA3.1) or the plasmid expressing human Nrf2. The luciferase activity was assayed after 24 h. The induced luciferase activity with co-expression with Nrf2 was not observed in a mutant NDP52 promoter in which all three ARE sites (−2,057, −1,023 and −94) were site-directly mutated, indicating these three sites of five ARE cis -acting elements are functional. Data shown are mean±s.d. of three independent experiments and were analysed using Student’s t -test. (* P <0.05; ** P <0.01; *** P <0.001). Full size image NDP52 facilitates the turnover of phosphorylated tau NDP52 has an LIR [28] and previous studies indicate that it functions as an autophagy adaptor recognizing ubiquitin-coated cytosolic bacteria or regulating Toll-like receptor signalling, but only in peripheral tissues [27] , [28] , [29] , [38] . Therefore, we examined the co-localization of NDP52 with LC3 in both primary cortical neurons and CN1.4 naive cells following transient transfection. Expression of NDP52 along with tau in primary cultured neurons resulted in prominent, NDP52-postive punctae in the soma of the neurons ( Supplementary Fig. 9a ). All the NDP52 punctae overlapped with autophagic vesicles as they were LC3 positive ( Supplementary Figs 9b,c and 10a,b ). In addition, when HEK 293-TN cells were transiently transfected with green fluorescent protein (GFP) or GFP-LC3, endogenous NDP52 was co-immunoprecipitated with GFP-LC3, but not with GFP alone ( Supplementary Fig. 11 ). The results indicate that NDP52 interacts with LC3 and probably plays a role in targeting client proteins to the autophagy pathway in neuronal cells. To further investigate the role of NDP52 in facilitating the turnover of phosphorylated tau in primary cultured neurons, we used recombinant lentiviruses expressing sh-RNA for Nrf2 or NDP52. When primary cortical neurons were transduced with sh-Nrf2, the levels of tau endogenously phosphorylated at Ser262/Ser356 [12E8] and Ser396/Ser404 [PHF1] were 1.5- and 1.9-fold increased, respectively, in comparison with what was observed in neurons transduced with sh-scramble ( Fig. 8a,b ). Transduction with sh-NDP52 resulted in 1.8- and 2.1-fold increases of tau phosphorylated at Ser262/Ser356 [12E8] and at Ser396/Ser404 [PHF1], respectively ( Fig. 8a,b ). A dramatic decrease in the levels of both wild-type tau and caspase-cleaved tau in HEK 293-TN cells was observed with co-expression of Nrf2 or NDP52 compared with the cells co-transfected with the mock plasmid, whereas co-expression of p62/SQSTM1 or the co-chaperone Bag2, which has been reported to be involved in the degradation of phosphorylated tau [7] , [23] , did not decrease tau levels ( Supplementary Fig. 12a,b ). In addition, a decrease in the intensity of endogenously phosphorylated tau immunostained with 12E8 or PHF1 antibody was observed in the primary neurons transduced with the recombinant lentivirus expressing NDP52 compared with those transduced with a control lentivirus in the presence of 150 mM trehalose, a disaccharide autophagy inducer [15] , [39] ( Fig. 8c–f and Supplementary Fig. 12c,d ). Together, these results suggest that NDP52 functions in facilitating the turnover of phosphorylated tau. 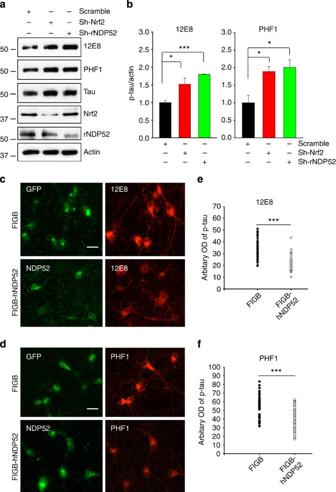Figure 8: NDP52 plays an important role in the clearance of phosphorylated tau. (a) Primary cortical neurons were transduced with lentivirus expressing sh-RNA for Nrf2 or rat NDP52 (rNDP52), or a scrambled sh-RNA at DIV 1, and were maintained until DIV 6. The levels of tau phosphorylated at Ser262/Ser356 and Ser396/Ser404 were analysed by immunoblotting using 12E8- and PHF1-specific antibodies, respectively. Total tau was detected with a polyclonal tau-specific antibody (Tau). The relative molecular masses (kDa) are indicated to the left of each blot. (b) Bar graph of the relative optical density of phosphorylated tau normalized to actin. Data shown are mean±s.e. of three independent experiments and were analysed using Student’st-test. (*P<0.05; ***P<0.001) (c,d) Primary cortical neurons were transduced with a control lentivirus (FIGB) or with one expressing human NDP52 (hNDP52) at DIV 1. To induce autophagy, trehalose (150 mM) was added at DIV 5 and the neurons incubated for 24 h (DIV 6). Primary cortical neurons were fixed with 4% paraformaldehyde, and stained with the 12E8 or PHF1 antibodies. Scale bar, 20 μm. The optical density of tau phosphorylated at Ser262/Ser356 (12E8). (e) and Ser396/Ser404 (PHF1) (f) in the soma of ~30 neurons randomly chosen was analysed with the ImageJ program. Data were analysed using Student’st-test (***P<0.001). Figure 8: NDP52 plays an important role in the clearance of phosphorylated tau. ( a ) Primary cortical neurons were transduced with lentivirus expressing sh-RNA for Nrf2 or rat NDP52 (rNDP52), or a scrambled sh-RNA at DIV 1, and were maintained until DIV 6. The levels of tau phosphorylated at Ser262/Ser356 and Ser396/Ser404 were analysed by immunoblotting using 12E8- and PHF1-specific antibodies, respectively. Total tau was detected with a polyclonal tau-specific antibody (Tau). The relative molecular masses (kDa) are indicated to the left of each blot. ( b ) Bar graph of the relative optical density of phosphorylated tau normalized to actin. Data shown are mean±s.e. of three independent experiments and were analysed using Student’s t -test. (* P <0.05; *** P <0.001) ( c , d ) Primary cortical neurons were transduced with a control lentivirus (FIGB) or with one expressing human NDP52 (hNDP52) at DIV 1. To induce autophagy, trehalose (150 mM) was added at DIV 5 and the neurons incubated for 24 h (DIV 6). Primary cortical neurons were fixed with 4% paraformaldehyde, and stained with the 12E8 or PHF1 antibodies. Scale bar, 20 μm. The optical density of tau phosphorylated at Ser262/Ser356 (12E8). ( e ) and Ser396/Ser404 (PHF1) ( f ) in the soma of ~30 neurons randomly chosen was analysed with the ImageJ program. Data were analysed using Student’s t -test (*** P <0.001). Full size image NDP52 interacts with tau through its SKICH domain To determine how NDP52 may facilitate the clearance of tau, we performed co-immunoprecipitation studies using HEK 293-TN cell lysates transfected with GFP or GFP-tau to determine whether NDP52 interacts with tau. Endogenous NDP52 protein co-immunoprecipitated with GFP-tau, but not with GFP alone ( Supplementary Fig. 13 ), indicating that NDP52 associates with tau. Human NDP52 consists of an amino-terminal skeletal muscle and kidney-enriched inositol phosphatase carboxyl homology (SKICH) domain (amino acids, 1–127), an intermediate coiled-coil (CC) domain (amino acids, 134–350) and a carboxy-terminal Lin11, Is1-1 and Mec-3 (LIM)-like (LIM-L) domain (amino acids, 395–446) [29] . To investigate which domain of NDP52 is required for the interaction with tau, co-immunoprecipitation studies were carried out using lysates prepared from CN1.4 naive cortical cells co-transfected with GFP-tau along with different human NDP52 constructs (full length, ΔSKICH, CC and ΔLIM-L) as shown in Fig. 9a . Full-length and the LIM-L domain-deleted construct of NDP52 co-immunoprecipitated with GFP-tau; however, ΔSKICH and CC domain-only constructs did not ( Fig. 9b ), suggesting that NDP52 interacts with tau through its SKICH domain. In CN1.4 mouse cortical cells [14] endogenous mouse NDP52, which does not have the LIM-like domain ( Fig. 9a ), also co-immunoprecipitated with tau (which was induced by treatment with doxycycline (1 μg ml −1 ) [14] ; Fig. 9c ). The results strongly indicate that NDP52 selectively interacts with tau through the SKICH domain. In addition, overexpression of human and mouse NDP52 in CN1.4 cortical cells decreased the levels of phosphorylated tau, but that of ΔSKICH did not, supporting the involvement of the SKICH domain in its binding to phosphorylated tau ( Fig. 9d and Supplementary Fig. 14 ). Further, knock down of mouse NDP52 using siRNA prevented the SFN-induced reduction of phosphorylated tau ( Fig. 9e ). Together, the results suggest that NDP52, including mouse NDP52 that does not have the LIM-L domain, interacts with tau via its SKICH domain, which is conserved in human, rat and mouse. It was previously reported that p62/SQSTM1 binding to non-ubiquitylated substrates facilitates autophagic clearance [40] . The LIM-L domain is known to bind specifically to ubiquitin chains of target molecules [28] . Considering the effect of mouse NDP52 on the degradation of phosphorylated tau, NDP52 probably plays a prominent role in the clearance of phosphorylated tau independent of ubiquitylation. 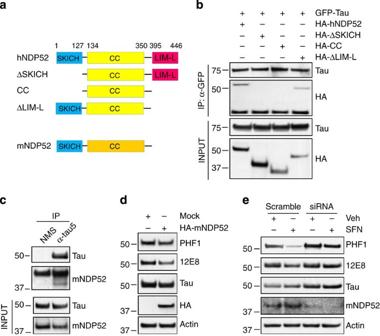Figure 9: The SKICH domain of NDP52 interacts with tau. (a) Schematic diagram of human NDP52, the domain-deleted constructs and mouse NDP52. (b) Naive cortical cells were co-transfected with the plasmids expressing HA-hNDP52 or HA-tagged domain-deleted mutants of human NDP52 together with GFP-tau. Twenty-four hours later, cell lysates were prepared and transfected tau was immunoprecipitated and blots probed for both the HA-hNDP52 constructs and GFP-tau. Homogenates (input) used for co-immunoprecipitation were analysed by immunoblotting using anti-HA or a polyclonal tau-specific antibody (Tau). (c) Stably transfected CN1.4 cortical cells were maintained in the presence of doxycycline (1 μg ml−1) to induce the expression of tau for 24 h. Homogenates from CN1.4 cortical cells were used for the co-immunoprecipitation of mouse NDP52 (mNDP52) using a Tau5 antibody. Co-precipitation of mNDP52 was examined by immunoblotting using anti-NDP52 antibody. Input of the homogenates used for co-immunoprecipitation was analysed by immunoblotting using anti-NDP52 or Tau antibody. (d,e) CN1.4 cortical cells were transfected with the mock or HA-mNDP52 plasmid (d) or with mNDP52 siRNA or scramble RNA as a control (e). The cells transfected with siRNA or scramble RNA were treated with SFN (10 μM) for 24 h. The levels of tau phosphorylated at Ser262/Ser356 and Ser396/Ser404 were analysed by immunoblotting using 12E8 and PHF1 antibodies, respectively. Total tau was detected with a polyclonal tau-specific antibody (Tau). The relative molecular masses (kDa) are indicated to the left of each blot. Figure 9: The SKICH domain of NDP52 interacts with tau. ( a ) Schematic diagram of human NDP52, the domain-deleted constructs and mouse NDP52. ( b ) Naive cortical cells were co-transfected with the plasmids expressing HA-hNDP52 or HA-tagged domain-deleted mutants of human NDP52 together with GFP-tau. Twenty-four hours later, cell lysates were prepared and transfected tau was immunoprecipitated and blots probed for both the HA-hNDP52 constructs and GFP-tau. Homogenates (input) used for co-immunoprecipitation were analysed by immunoblotting using anti-HA or a polyclonal tau-specific antibody (Tau). ( c ) Stably transfected CN1.4 cortical cells were maintained in the presence of doxycycline (1 μg ml −1 ) to induce the expression of tau for 24 h. Homogenates from CN1.4 cortical cells were used for the co-immunoprecipitation of mouse NDP52 (mNDP52) using a Tau5 antibody. Co-precipitation of mNDP52 was examined by immunoblotting using anti-NDP52 antibody. Input of the homogenates used for co-immunoprecipitation was analysed by immunoblotting using anti-NDP52 or Tau antibody. ( d , e ) CN1.4 cortical cells were transfected with the mock or HA-mNDP52 plasmid ( d ) or with mNDP52 siRNA or scramble RNA as a control ( e ). The cells transfected with siRNA or scramble RNA were treated with SFN (10 μM) for 24 h. The levels of tau phosphorylated at Ser262/Ser356 and Ser396/Ser404 were analysed by immunoblotting using 12E8 and PHF1 antibodies, respectively. Total tau was detected with a polyclonal tau-specific antibody (Tau). The relative molecular masses (kDa) are indicated to the left of each blot. Full size image NDP52 decreases sarkosyl-insoluble tau in AD cases We performed co-immunoprecipitation studies using lysates prepared from human AD cerebral cortex. Endogenous, human NDP52 protein co-immunoprecipitated when the phosphorylated tau antibodies 12E8 or PHF1 were used, but not when the phospho-independent Tau5 antibody was used ( Fig. 10a,b ). These results would suggest that NDP52 may more efficiently interact with phosphorylated forms of tau than with tau that is not pathologically phosphorylated. 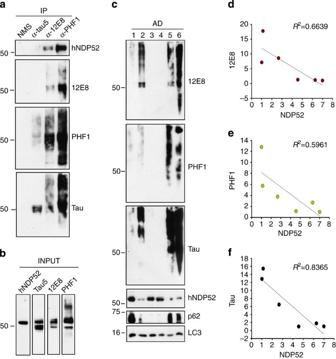Figure 10: The amount of sarkosyl-insoluble human tau is inversely proportional to that of human NDP52. (a) Homogenates from cerebral cortical tissue of a diagnosed AD case were used for the co-immunoprecipitation of human NDP52 (hNDP52) using a Tau5, 12E8 or PHF1 antibody. (b) Homogenates used for co-immunoprecipitation inawere analysed by immunoblotting using anti-NDP52, Tau5, 12E8 or PHF1 antibody. (c) Cerebral cortical tissues from diagnosed AD cases were separated into sarkosyl-soluble and insoluble fractions. The levels of total tau and tau phosphorylated at Ser262/Ser356 and Ser396/Ser404 in the sarkosyl-insoluble fractions were analysed by immunoblotting using 12E8 and PHF1 antibodies, respectively. Samples were also immunoblotted with a polyclonal to total tau (Tau) antibody. The levels of hNDP52, p62/SQSTM1 and LC3 in the sarkosyl insoluble fractions also were examined by immunoblotting. The relative molecular masses (kDa) are indicated to the left of each blot. (d–f) The regression graphs show the relative amount of tau phosphorylated at Ser262/Ser356 (12E8) (d), at Ser396/Ser404 (PHF1) (e) or total tau (f) compared to hNDP52 present in the sarkosyl-insoluble fractions. Figure 10: The amount of sarkosyl-insoluble human tau is inversely proportional to that of human NDP52. ( a ) Homogenates from cerebral cortical tissue of a diagnosed AD case were used for the co-immunoprecipitation of human NDP52 (hNDP52) using a Tau5, 12E8 or PHF1 antibody. ( b ) Homogenates used for co-immunoprecipitation in a were analysed by immunoblotting using anti-NDP52, Tau5, 12E8 or PHF1 antibody. ( c ) Cerebral cortical tissues from diagnosed AD cases were separated into sarkosyl-soluble and insoluble fractions. The levels of total tau and tau phosphorylated at Ser262/Ser356 and Ser396/Ser404 in the sarkosyl-insoluble fractions were analysed by immunoblotting using 12E8 and PHF1 antibodies, respectively. Samples were also immunoblotted with a polyclonal to total tau (Tau) antibody. The levels of hNDP52, p62/SQSTM1 and LC3 in the sarkosyl insoluble fractions also were examined by immunoblotting. The relative molecular masses (kDa) are indicated to the left of each blot. ( d – f ) The regression graphs show the relative amount of tau phosphorylated at Ser262/Ser356 (12E8) ( d ), at Ser396/Ser404 (PHF1) ( e ) or total tau ( f ) compared to hNDP52 present in the sarkosyl-insoluble fractions. Full size image Cortical tissues from AD cases ( Supplementary Table 1 ) were then separated into soluble, sarkosyl-soluble and sarkosyl-insoluble fractions. No correlation between the amount of phosphorylated tau and the amount of NDP52 was observed in the soluble and sarkosyl-soluble fractions. In contrast, the amount of total tau, as well as tau phosphorylated at Ser262/Ser356 [12E8] or a Ser396/Ser404 [PHF1], in the sarkosyl-insoluble fractions was inversely proportional to that of human NDP52 ( Fig. 10c–f ). This result indicates that NDP52 may prevent the aggregation of tau through the clearance of phosphorylated tau. Tau is normally an abundant soluble neuronal protein; however, in AD tau becomes inappropriately phosphorylated and eventually accumulates as neurofibrillary tangles [1] , [2] , [3] . There is increasing evidence that the accumulation of soluble, but pathologically phosphorylated and oligomerized tau is probably a toxic event compromising neuronal function [41] , [42] , [43] . Hence, the strategy of promoting the clearance of pathological tau in AD has been proposed as a therapeutic approach [2] , [4] . In this context, understanding the mechanisms involved in selectively directing pathological, phosphorylated forms of tau to a degradative pathway is of significance. In this study, we found that NDP52, which is an autophagy adaptor that contains an LIR [28] , is induced by Nrf2 and may play an important role in directing tau, particularly phosphorylated tau, to the autophagic degradative pathway. The expression of p62/SQSTM1 is induced by the activation of Nrf2 (ref. 22 ). Since the accumulation of hyperphosphorylated tau was observed in the brains of p62/SQSTM1 (−/−) mice [23] , we postulated that p62/SQSTM1 might be involved in the Nrf2-mediated degradation of phosphorylated tau ( Figs 1 and 3 ). Although a 1.9-fold decrease in the mRNA levels for p62/SQSTM1 was observed in Nrf2 (−/−) mice, the protein level of p62/SQSTM1 was not changed compared with wild-type mice ( Fig. 6b,c ). In addition, the protein levels of Keap1 (Kelch-like ECH-associated protein 1), an adaptor protein for Cul3-based ubiquitin E3 ligase complex for Nrf2, showed no difference between Nrf2 (−/−) and wild-type mice ( Fig. 6c ), indicating that the activity of p62/SQSTM1 in Nrf2 (−/−) mice may not be different from that of wild-type mice. Although we could not exclude completely a role for p62/SQSTM1 as an autophagy adaptor for phosphorylated or misfolded tau in our models, our data strongly indicate that NDP52 is probably a primary autophagy adaptor that is facilitating degradation of phosphorylated tau. Activation of Nrf2 in response to SFN treatment resulted in the induction of NDP52 at both the message and protein level in the neuronal models used in this study ( Fig. 6a,d,e and Supplementary Fig. 7 ). In Nrf2 (−/−) mice the expression levels of p62/SQSTM1 and NDP52 were reduced 1.9- and 7.8-fold, respectively, indicating that the expression of NDP52 is more dependent on Nrf2 activity than that of p62/SQSTM1 ( Fig. 6b ). Since the degradation of Keap1 is dependent on the activity of p62/SQSTM1 (ref. 21 ), it is plausible that Keap1, a cytosolic inhibitor of Nrf2, would accumulate in p62/SQSTM1 -knockout mice, thus blocking the activation of Nrf2. Therefore, it can be speculated that the accumulation of phosphorylated tau observed in p62/SQSTM1 -knockout mice [23] could be in part due to a decreased expression of NDP52 by means of reduced Nrf2 activity. A complex consisting of the E3 ligase CHIP (C terminus of Hsp70-interacting protein) in conjunction with several chaperones probably plays a role in maintaining tau in a functional conformation or directing it towards the degradation machinery [8] , [44] , [45] , [46] . In this paradigm, inhibition of the chaperone function of Hsp90 results in CHIP/Hsp70-mediated ubiquitylation of tau, and subsequent degradation [45] , [47] . Interestingly, Hsp90 inhibition did not affect the levels of tau phosphorylated at S262/S356 [12E8] [47] , and CHIP was unable to bind and ubiquitylate tau phosphorylated at S262/S356 [12E8] site as well [8] , indicating that tau phosphorylated at S262/S356 [12E8] site may not be recognized by this chaperone network. In this present study, by contrast, Nrf2 activation or NDP52 overexpression in neurons reduced the levels of tau phosphorylated at S396/S404 [PHF1] and/or S262/S356 [12E8] site(s) ( Figs 3 , 8c–f and 9d and Supplementary Figs 3a–c and 12 ). Therefore, it can be suggested that the chaperone system and NDP52-mediated system may be complimentary in facilitating the clearance of different forms of tau. Previously, NDP52 had been identified primarily in peripheral tissues as an innate immune autophagy receptor involved in the clearance of cytosolic bacteria [27] , [28] , [38] . Our results of these studies demonstrate for the first time that NDP52 is in the brain ( Figs 6 and 10 and Supplementary Fig. 8 ) and expressed in neurons ( Figs 6 , 8 and 9 ), and is strongly regulated by Nrf2 ( Figs 6 and 7 and Supplementary Fig. 8c,d ). Further, we provide unique insight into NDP52 as an autophagy adaptor protein in the clearance of pathologic, phosphorylated tau in neurons ( Figs 8 , 9 , 10 and Supplementary Fig. 12 ). In previous studies, the hippocampal expression of Nrf2 or its activation with Nrf2 activators such as SFN, curcumin and α-lipoic acid in murine AD models significantly improved learning and memory retention compared with untreated animals [33] , [34] . It is therefore plausible that NDP52 induced by Nrf2 could play a role in the improvement of AD symptoms through the clearance of pathological, phosphorylated tau. Thus, the pre-emptive activation of Nrf2 through the use of Nrf2 activators could be a possible therapeutic strategy for delaying the onset and slowing the progression of AD. Plasmids and reagents Tau5, PHF1 (phospho-Ser396/404) and 12E8 (phospho-Ser262/356) antibodies were kindly provided by Dr L. Binder, Dr P. Davies and Dr P. Seubert, respectively. Polyclonal tau (A0024) antibody was purchased from Dako. Anti-Nrf2 (ab31163) antibody was obtained from Abcam. Anti-NDP52 (ab68588) antibody for human and rat NDP52 was purchased from Abcam, while the one (H00010241-B01P) used for mouse NDP52 was from Novus Biologicals [48] . Anti-p62/SQSTM1 (BML-PW9860), Keap1 (10503-2-AP), Hsp70 (ADI-SPA-757), GFP (11-814-460-001) and actin (MAB1501) antibodies were purchased from Biomol, Proteintech, Assay Designs, Roche and Chemicon, respectively. Anti-HA (2367), beclin-1 (3495), histone (12349) and Myc (9B11) (2276) were obtained from Cell Signaling Technology. The pEGFP-human NDP52 plasmid was generously provided by Dr J. Kendrick-Jones. The haemagglutinin (HA)-tagged human NDP52 (HA-hNDP52), SKICH domain-deleted HA-hNDP52 (ΔSKICH), LIM-like domain-deleted HA-hNDP52 (ΔLIM-L) and both SKICH and LIM-like domain-deleted HA-hNDP52 (CC) were gifts from by Dr T. Into. The pcDNA3-Myc3-human Nrf2 plasmid was obtained from Addgene. The lentiviral vector expressing human NDP52 was constructed by subcloning the amplified gene into the AgeI and BamHI sites of the lentiviral expression plasmid, FIGB (a generous gift from Dr C Proschel). The lentiviral vectors expressing short hairpin RNA for scrambled, Nrf2 and NDP52 ( Supplementary Table 2 ) were constructed by subcloning the cassette containing the H1 promoter and short hairpin RNA sequence from pSuper-GFP/neo (OligoEngine) into the HpaI and PacI sites of the lentiviral plasmid FG12 (Addgene). The vectors pVSV-G (encoding the viral envelope) and psPAX2 (encoding gag-pol) were from Addgene. The human promoter of NDP52 was amplified from human genomic DNA (Affymetrix), and cloned to the SacI and EcoRV sites of the pGL4.14-Luc reporter plasmid (Promega, E6691). The thymidine kinase-renilla plasmid (E224A) was from Promega. The ARE-Luc reporter plasmid was kindly provided by Dr MO Leonard. The plasmid expressing GFP-tau was constructed by subcloning the human tau gene into the HindIII and BamHI sites of the pEGFP-C1 plasmid (Clontech, 6084-1). The preparation of the plasmids expressing wild-type human tau (T4) and caspase-cleaved tau (T4C3) are described in the previous studies [49] , [50] . In brief, T4 was subcloned into the mammalian expression vector, pcDNA 3.1(−) (Invitrogen) at the EcoRI and KpnI sites. T4 in pcDNA 3.1(−) was then used as a template and PCR was performed with forward primer 5′-CGC GGA TCC GCG ATG GCT GAG CCC CGC CAG GAG TTC-3′ and reverse primer 5′-CTG CTC TAG AGC ATC AGT CTA CCA TGT CGA TGC TGC CGG TGG-3′ to remove the last 20 amino acids of tau and subcloned into the BamHI and XbaI sites of pcDNA3.1(+). GFP-LC3 was prepared by using RNA extracted from naive CN1.4 cells, creating complementary DNA by reverse transcription using Superscript III (Invitrogen, 12574030), followed by PCR and insertion into the EcoRI site of pEGFP-C1 as described previously [14] . YFP-Bag2 and Myc-p62/SQSTM1 were gifts from by Dr KS Kosik and Dr T Johansen, respectively. The plasmid expressing HA-Bag2 was prepared by subcloning the mouse Bag2 gene into the KpnI and EcoRI sites of the pHM6 plasmid (Roche). The plasmids expressing mCherry-hNDP52 and mCherry-mNDP52 were constructed by subcloning human NDP52 and mouse NDP52 gene into BamHI and EcoRI sites and EcoRI and XhoI sites of the pmCherry plasmid (Clontech, 632524), respectively. All constructs were confirmed by sequencing. SFN (574215), trehalose (625625), epoxomicin (324800) and bafilomycin A1 (196000) were purchased from Calbiochem. 3-MA (M9281) and CQ (C6628) were from Sigma. Mice The Nrf2 -knockout (−/−) mice on a C57BL/6J background were generously supplied by Dr M Yamamoto [51] via the RIKEN BioResource Center, Tsukuba, Japan. Wild-type C57BL/6J mice were purchased from Jackson Laboratories. Information about the age and sex of the mice used are given in the appropriate figure legends. All animal protocols for this study were approved by the University Committee on Animal Research of the University of Rochester. Human samples Human brain tissues (0.2 g) were homogenized in 1 ml of ice-cold soluble buffer (0.1 M MES (pH 7.0), 1 mM EDTA, 0.5 mM MgSO 4 , 1 M sucrose) containing 1 mM NaF, 1 mM Na 3 VO 4 , 1 mM phenylmethyl sulphonyl fluoride and 10 μg ml −1 each of aprotinin, leupeptin and pepstatin. The homogenates were cleared by centrifugation at 50,000 g for 20 min at 4 °C, and the supernatants were collected as soluble fractions. To prepare the sarkosyl-insoluble fraction, the pellets were resuspended in RAB buffer (100 mM MES (pH6.8), 10% sucrose, 2 mM EGTA, 0.5 mM MgSO 4 , 500 mM NaCl, 1 mM MgCl 2 , 10 mM NaH 2 PO 4 , 20 mM NaF) containing 1% N -lauroylsarcosine (Sarkosyl) with protease inhibitors, vortexed for 1 min at room temperature, incubated at 4 °C overnight, and then centrifuged at 200,000 g for 30 min at room temperature. The supernatants were collected as sarkosyl-soluble fractions, and the pellets, sarkosyl-insoluble fractions, were resuspended in 1 × SDS protein loading buffer and incubated in 95 °C for 5 min. Pre-existing AD brain samples were obtained from the University of Rochester Medical Center Brain Bank. The protocol was designated as exempt (exemption number 4) by the Institutional Review Board at the University of Rochester as it was a retrospective study of autopsy specimens that were pre-existing and de-identified. Cell culture Immortalized mouse cortical CN1.4 naive cells [52] (a gift from Dr Campagnoni) and CN1.4 cells that we engineered to inducibly express full-length tau in the presence of the tetracycline derivative doxycycline [14] were cultured in DMEM supplemented with 5% fetal bovine serum (FBS), 0.1% gentamicin, 4 mM glutamine, and 10 units ml −1 penicillin and 100 units ml −1 streptomycin at 33 °C in a humidified atmosphere containing 5% CO 2 . In this study, cells were treated with doxycycline at a concentration of 1 μg ml −1 for 24 h to induce tau expression. HEK293-TN and SH-SY5Y cells were grown in DMEM supplemented with 10% FBS, 10 units ml −1 penicillin and 100 units ml −1 streptomycin. Cells were maintained at 37 °C in a humidified atmosphere containing 5% CO 2 . Primary cell culture and transduction Primary cortical neuronal cultures from rat embryonic forebrain were prepared and maintained as described previously with modification [53] . In brief, whole brains were removed from E18 rats. The cortices were dissected, treated with 0.05% trypsin at 37 °C for 30 min and gently triturated with a fire polished glass Pasteur pipette. Dissociated cells were plated onto 6-well plates or glass coverslips in 12-well plates coated with poly- D -lysine (40 μg ml −1 , Millipore, A-003-E) in MEM (Invitrogen, 11090) containing 5% FBS, 20 mM glucose, 2 mM glutamine in the incubator at 37 °C in a humidified atmosphere containing 5% CO 2 . Five hours after plating, medium was replaced with Neurobasal medium (Invitrogen, 21103-049) supplemented with 0.5 mM glutamine and 2% B27 (Invitrogen, 17504-044). One-half of the medium was replaced with the fresh, complete Neurobasal medium every 3 day. On DIV (day in vitro ) 1, 20 μl of virus solution was added directly to the media on the neurons cultured in 6-well plates or 10 μl of virus solution in 12-well plates, and the medium was replaced after 12 h. Experiments were performed on DIV 6–7. Lentivirus production HEK 293-TN cells (a generous gift from Dr C Proschel) were transfected with the lentiviral plasmid/psPAX2/pVSV-G using Lipofectamine 2000 (Invitrogen, 11668-019). Twelve hours post transfection, media was replaced with DMEM supplemented with 1% FetalcloneII, and the cells were incubated at 33 °C in a humidified atmosphere containing 5% CO 2 . Seventy-two hours later, the media was collected, spun at 800 g for 10 min at room temperature and the resulting supernatant was then centrifuged at 60,000 g for 2 h at 4 °C. The pellet was resuspended in 500 μl sterile PBS containing 0.1% BSA per 100 mm dish, and the lentiviral solution was used immediately. Protein kinase assay Mouse brain tissue was homogenized in lysis buffer (50 mM Tris–HCl (pH 7.9), 100 mM NaCl, 10 mM MgCl 2 , 1 mM DTT) containing 0.1% NP-40 and protease inhibitors. Proteins were extracted on ice with periodic vortexing for 30 min, and lysates were cleared by centrifugation at 10,000 g for 10 min at 4 °C. Ten micrograms of lysates was incubated with 2 μg of glutathione S -transferase (GST)-tau protein at 37 °C for 30 min in buffer consisting of 25 mM Tris–HCl (pH 7.4), 10 mM MgCl 2 , 1 mM EGTA, 1 mM DTT, 0.2 mM NaF, 0.1 mM Na 3 VO 4 , 1 μg ml −1 aprotinin, 10 μM dibutyryl-cyclic AMP (Tocris, 1141) and 10 nM okadic acid without or with 1 mM ATP. The reaction was stopped by the addition of 1 × SDS-sample loading buffer and boiling at 95 °C for 5 min. Proteins were separated by SDS–PAGE and immunoblotted as described below. Phosphatase assay Phosphatase activity of mouse brain tissues was quantified using the serine/threonine phosphatase assay system (Promega, V2460) by measuring the dephosphorylation of a phosphopeptide, RRA(pT)VA. In brief, mouse brain tissues were homogenized in the phosphatase storage buffer (10 mM Tris–HCl (pH 7.4), 150 mM NaCl, 1 mM EDTA, I mM EGTA, 0.5% NP-40) containing protease inhibitors. Proteins were extracted on ice with periodic vortexing for 30 min, and lysates were cleared by centrifugation at 10,000 g for 10 min at 4 °C. Two hundred microlitres of supernatants was passed through Sephadex G-25 column to remove the residual phosphate in the supernatants. Two microlitres of samples was incubated with 100 μM of phosphopeptide (RRA(pT)VA) at 37 °C for 30 min in buffer consisting of 250 mM imidazole (pH 7.2), 1 mM EGTA, 50 mM MgCl 2 , 5 mM NiCl 2 , 250 μg ml −1 calmodulin and 0.1% β-mercaptoethanol without or with 20 nM okadaic acid. To terminate the reaction, 50 μl of molybdate dye with additive mixture was added to the mixture. The mixture was incubated for 10 min at room temperature to allow colour development. Absorbance was measured at A 600 using the Synergy HT plate reader (BioTek). Phosphate released was determined by comparing absorbance with a standard phosphate curve. PP2A activity was defined as the activity inhibited by the addition of 20 nM okadaic acid to the phosphatase reaction mixture. ChIP assay ChIP was performed following the protocol from Upstate (Temecula, CA). In brief, cells were treated with 1% formaldehyde at 37 °C for 10 min to cross-link chromatin and lysed with SDS lysis buffer containing protease inhibitors. Then, the cell extracts were sonicated to shear DNA and immunoprecipitated using an Nrf2 (1:100) or histone (1:100) antibody. Immunoprecipitates containing protein–DNA complexes were washed according to the instruction. To reverse cross-links, 20 μl of 5 M NaCl was added to the eluates (500 μl) and heated at 65 °C for 4 h. The eluates were then treated with 10 μl of proteinase K (20 μg ml −1 ) in a buffer containing 20 μl of 1 M Tris–HCl (pH 6.5) and 10 μl of 0.5 M EDTA, and incubated at 45 °C for 1 h. DNA was recovered by phenol/chloroform extraction and ethanol precipitation. To analyse ChIP products, PCR primers ( Supplementary Table 3 ) were designed to flank ARE sequence in the human NDP52 promoter. PCR was performed with samples of ChIP DNAs for 35 cycles of denaturation at 97 °C for 30 s, annealing at 56 °C for 30 s and extension at 72 °C for 1 min. siRNA transfection For knockdown of endogenous mouse NDP52, mouse NDP52-specific siRNA or scrambled RNA as a control ( Supplementary Table 4 ) was mixed with Oligofectamine (Invitrogen, 12252-011) in serum-free Opti-MEM medium for 15 min. The mixture was loaded onto CN1.4 cortical neurons [14] following exchange of the culture medium for serum-free DMEM medium. After 4 h, FBS was added up to 5% and maintained at 33 °C in a humidified atmosphere containing 5% CO 2 for 24 h. The human beclin-1-specific siRNA (6222) was purchased from Cell Signaling Technology. Transient transfection and luciferase assays Cells were transiently transfected with human NDP52 promoter cloned to the reporter plasmid pGL4.14-Luc (Promega) together with the thymidine kinase-renilla plasmid using Lipofectamine 2000 (Invitrogen). The total amount of DNA used for each well or plate was normalized with the relevant mock vectors. Luciferase activity was measured using the luciferase assay system (Promega, E2920) and a luminometer (Turner Designs). Transfection efficiency was normalized with renilla activity. Immunoblotting Cells were washed once with PBS and lysed with modified RIPA buffer (10 mM Tris–HCl (pH 7.4), 150 mM NaCl, 1 mM EGTA, 1% NP-40, 0.25% sodium deoxycholate, 0.1% SDS) containing 1 mM NaF, 1 mM Na 3 VO 4 , 1 mM phenylmethyl sulphonyl fluoride and 10 μg ml −1 each of aprotinin, leupeptin and pepstatin. Proteins were extracted on ice with periodic vortexing for 30–40 min, and lysates were cleared by centrifugation at 10,000 g for 10 min at 4 °C, and the supernatants were used for immunoblotting following boiling in 1 × SDS-sample loading buffer for 5 min. For analysis, samples (10–50 μg protein) were separated on 8, 10 or 12% SDS–PAGEs followed by transfer to nitrocellulose membranes (Bio-Rad) and immunoblotting with the indicated antibodies: Tau5 (1:25,000), PHF1 (1:5,000), 12E8 (1:5,000), polyclonal tau (1:500,000), Nrf2 (1:2,000), NDP52 (1:2,000), mouse NDP52 (1:500), p62/SQSTM1 (1:5,000), Keap1 (1:2,500), Hsp70 (1:5,000), GFP (1:5,000), actin (1:50,000), HA (1:1,000), beclin-1 (1:1,000) and Myc (9B11) (1:1,000) antibodies. Blots were developed with chemiluminescence. All protein concentrations were determined using the bicinchoninic acid method (Sigma). Full blots are shown in Supplementary Fig. 15 . Immunoprecipitation Human brain tissue (0.2 g) or cells were lysed in NP-40 lysis buffer (0.5% NP-40, 10 mM Tris–HCl (pH 8.0), 150 mM NaCl, 10 mM sodium pyrophosphate, 1 mM EDTA) containing 1 mM NaF, 1 mM Na 3 VO 4 and protease inhibitors. Equal amounts of lysates were incubated with 2 μg of antibodies pre-conjugated with sheep anti-mouse magnetic beads (DYNAL, Invitrogen, 110-31) for 3 h on a rotational shaker at 4 °C. After overnight incubation at 4 °C, the beads were washed with three changes of NETN wash buffer (0.1% NP-40, 50 mM Tris–HCl (pH 8.0), 150 mM NaCl, 1 mM EDTA) and boiled in 1 × SDS-sample loading buffer for 5 min. Proteins were separated by SDS–PAGE and immunoblotted as described above. Immunohistochemical staining Brain slices (30 μm) prepared from mouse brains fixed with 4% paraformaldehyde were washed three times using PBS to remove cryoprotectant, and incubated in TBS containing 10% normal goat serum (NGS) and 0.4% Triton X-100 for 1 h at room temperature. To detect phosphorylated tau, the sections were incubated with a 12E8 (1:500) or PHF1 (1:600) antibody containing 5% NGS and 0.1% Triton X-100 in TBS (incubation solution) for overnight at 4 °C. On the next day, slices were incubated for 1 h at room with Alexa Fluro 594-conjugated secondary antibody (1:500, Invitrogen) followed by three washes with the incubation solution. For the immunostaining of primary cortical neurons grown on coverslips (18 mm), neurons were fixed with 4% paraformaldehyde in PBS, followed by a permeabilization with TBS containing 0.2% Triton X-100 for 30 min and a pre-blocking with the incubation solution containing 5% NGS and 0.1% Triton X-100 in TBS for 1 h at room temperature. To detect phosphorylated tau, coverslips were incubated overnight at 4 °C with a 12E8 (1:1,000) or PHF1 (1:2,000) antibody in incubation solution, followed by incubation with the secondary antibody bound to Alexa 594 fluorophore (Invitrogen). The coverslips were mounted on the glass slides with ProLong gold antifade reagent (Invitrogen, P36935) following three washes with TBS. Images were photographed using a fluororescence microscope (Carl Zeiss AX10). Quantitative real-time PCR For the synthesis of cDNA, total RNA was isolated using Trizol (Invitrogen) according to the manufacture’s protocol. cDNA was generated using 2 μg of RNA, oligo-dT and Superscript III (Invitrogen). qRT–PCR was performed using the SYBR Green real-time PCR master mix (Invitrogen, 4344463) on a Bio-Rad IQ5 Real-Time PCR Detection System. Each reaction consisted of 10 μl of cDNA product from the diluted reverse transcription reaction (30 × ), 2.5 μM of primers (forward and reverse, Supplementary Table 5 ), 12.5 μl of SYBR Green real-time PCR master mix. The reactions were incubated in a 96-well plate at 95 °C for 5 min, followed by 45 cycles of 95 °C for 15 s, 60 °C for 20 s and 72 °C for 40 s. After the reactions were completed, the threshold was manually set and the threshold cycle was automatically recorded. The threshold cycle is defined as the fractional cycle number at which the fluorescence signal passes the fixed threshold. All reactions were run in three replicates for each sample. Resazurin assay The cell viability was determined by monitoring conversion of resazurin to a fluorescent product resorufin. Twenty-four hours after treatment of neurons with SFN or tBHQ in 24-well plates, resazurin at a final concentration of 400 μM was added to the media. Two hours after incubation, resorufin fluorescence was measured using the Synergy HT plate reader (BioTek) with excitation at 540 nm and emission at 590 nm. Results are presented as a percent of control cells. RT–PCR For the synthesis of cDNA, total RNA was isolated using Trizol (Invitrogen) according to the manufacture’s protocol. cDNA was synthesized using 2 μg of RNA with EcoDry premix (Clontech, 639543). Mouse NDP52 gene was amplified using the PCR premix (Bioneer, Korea) following the addition of 1 μl of cDNA product and 1 μM of primers (forward and reverse, Supplementary Table 6 ) on a PCR machine (Applied Biosystems). The reaction tubes were incubated at 96 °C for 5 min, followed by 35 cycles of 96 °C for 30 s, 58 °C for 30 s and 72 °C for 45 s. The PCR products were analysed by the agarose gel (1.2%) electrophoresis. How to cite this article: Jo, C. et al. Nrf2 reduces levels of phosphorylated tau protein by inducing autophagy adaptor protein NDP52. Nat. Commun. 5:3496 doi: 10.1038/ncomms4496 (2014).